Tension on the linker gates the ATP-dependent release of dynein from microtubules Cytoplasmic dynein is a dimeric motor that transports intracellular cargoes towards the minus end of microtubules (MTs). In contrast to other processive motors, stepping of the dynein motor domains (heads) is not precisely coordinated. Therefore, the mechanism of dynein processivity remains unclear. Here, by engineering the mechanical and catalytic properties of the motor, we show that dynein processivity minimally requires a single active head and a second inert MT-binding domain. Processivity arises from a high ratio of MT-bound to unbound time, and not from interhead communication. In addition, nucleotide-dependent microtubule release is gated by tension on the linker domain. Intramolecular tension sensing is observed in dynein’s stepping motion at high interhead separations. On the basis of these results, we propose a quantitative model for the stepping characteristics of dynein and its response to chemical and mechanical perturbation. Cytoplasmic dynein is responsible for nearly all microtubule (MT) minus-end-directed transport in eukaryotes [1] . In interphase cells, dynein transports membrane-bound organelles and vesicles [1] . During mitosis, dynein positions the spindle [2] , focuses the MTs into poles [3] and regulates the spindle assembly checkpoint [4] . Impaired dynein function has been implicated in motor neuron degeneration [5] , lissencephaly, and primary ciliary dyskinesia [6] . The ability of dynein to move processively and maintain contact with the MT is thought to be essential for its cellular roles, and small perturbations in dynein processivity were implicated in motor neuron degeneration [7] . However, the mechanism underlying these properties is not well understood. Dynein’s structure is unique among cytoskeletal motors. The ~350 kDa dynein motor domain (head) is much larger than that of kinesin or myosin, and contains six AAA+ subunits arranged in a hexameric ring ( Fig. 1a ) [7] , [8] , [9] . Unlike kinesin, whose MT binding and ATPase sites are part of the same globular domain, dynein’s MT-binding domain (MTBD) is located at the end of a coiled-coil stalk [10] . The linker, a helical bundle extending from the ring, is thought to be the mechanical element of dynein motility [9] , [11] , [12] . The linker shifts its position relative to the ring as a function of the nucleotide state of AAA1 (ref. 12 ) and its conformation correlates with MT affinity [13] . The linker makes multiple contacts with the ring, and disruption of these contacts reduces catalytic activity [7] , [8] . Therefore, apart from functioning as a lever arm, the linker may also play a regulatory role in the nucleotide hydrolysis cycle. 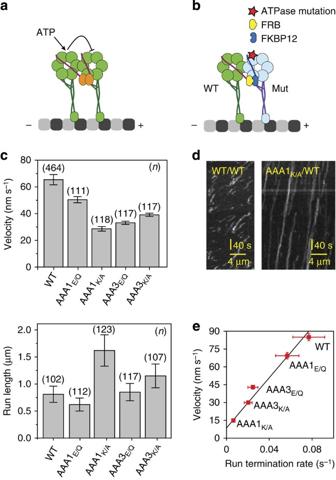Figure 1: Motile properties of heterodimeric dynein constructs bearing a single ATPase mutation. (a) Dynein monomers truncated at the N-terminal tail are dimerized through an N-terminal GST tag (orange). The nucleotide-gating model requires the ATPase cycles of the two heads to be kept out of phase. (b) A schematic (right) of FRB-FKBP12 dynein heterodimer on a MT. One of the heads (blue) contains specific mutations at an ATPase site. (c) Average velocity (±s.e.m.) and run length (±95% CI) of TMR-labelled dynein motors at 2 mM ATP. One WT monomer is dimerized with a partner carrying the indicated ATPase mutation. (d) Kymographs showing the processive movement of WT/WT and AAA1K/A/WT motors. (e) Plot of velocity versus run termination rate for the indicated heterodimers shows a linear relationship (black line). Figure 1: Motile properties of heterodimeric dynein constructs bearing a single ATPase mutation. ( a ) Dynein monomers truncated at the N-terminal tail are dimerized through an N-terminal GST tag (orange). The nucleotide-gating model requires the ATPase cycles of the two heads to be kept out of phase. ( b ) A schematic (right) of FRB-FKBP12 dynein heterodimer on a MT. One of the heads (blue) contains specific mutations at an ATPase site. ( c ) Average velocity (±s.e.m.) and run length (±95% CI) of TMR-labelled dynein motors at 2 mM ATP. One WT monomer is dimerized with a partner carrying the indicated ATPase mutation. ( d ) Kymographs showing the processive movement of WT/WT and AAA1 K/A /WT motors. ( e ) Plot of velocity versus run termination rate for the indicated heterodimers shows a linear relationship (black line). Full size image The mechanism of dynein motility also differs significantly from other motors. Processive kinesin and myosins walk hand-over-hand [14] , [15] , [16] , [17] , in which the heads are coordinated and take alternating steps. In contrast, dynein heads step independently of their partner [18] , [19] . It remains unknown what prevents both heads from releasing simultaneously in the absence of strict interhead coordination. Established views of motor processivity propose that, to keep the two heads out of phase, a chemical or structural change in one head must be gated until the other head proceeds through a critical step in its cycle. Several mechanisms have been proposed for motor gating [20] . When two heads are bound to the MT, the motor may experience tension through the linker domains. Interhead tension may accelerate the release of the rear head or inhibit nucleotide binding to the front head [21] , [22] . Reducing tension through peptide insertions affects kinesin velocity and efficiency of converting ATP hydrolysis into motion [23] , [24] , and decreases myosin VI processivity [25] . Alternatively, the nucleotide cycle of one head may allosterically affect that of the other head, so one head stays tightly bound to MT until the other head detaches from the MT and takes a step [26] . In the case of AAA+ enzymes, the rings may also directly interact with each other [27] . Indeed, stacking interactions between the rings were observed in electron microscopy images of axonemal dynein [28] . In this study, we tested the structural and catalytic requirements of dynein processivity. To construct a minimally processive dynein motor, we altered the mechanical and catalytic properties of Saccharomyces cerevisiae dynein and tested their role in motility at a single molecule level. We find that processivity minimally requires a single active monomer and a tether retaining only the MTBD. The degree of processivity is determined by the MT affinity of the tether. Dynein processivity does not require any of these gating strategies to prevent simultaneous dissociation of both heads from MT. However, dynein remains partially gated at high interhead separations. To test whether the mechanism of this conditional gating is due to linker tension, we pulled dynein monomers through their C terminus or the N-terminal linker using an optical trap under different nucleotide conditions. Remarkably, exerting tension on the linker fully abolishes the ATP-dependent MT release of the motor. High-resolution multicolour tracking of a heterodimeric dynein with one active and one inactive head showed that the stepping rate of an active head is high when it is positioned close to its inactive partner, but remains low when it is positioned apart. The results reveal a critical role of the linker in gating dynein stepping behaviour and suggest that dynein steps in a tension-dependent manner at high interhead separations. Using our experimental results, we developed a computational model for the dynein stepping mechanism in the absence of tight interhead communication. Does dynein processivity require nucleotide gating? A nucleotide-gating mechanism proposes that the nucleotide states of the heads remain out of phase such that one head remains tightly bound to the MT as the other head releases and takes a step. The model requires both heads to be catalytically active and able to change their MT affinity in a nucleotide-dependent manner ( Fig. 1a ). To test the predictions of this model, we disrupted ATP binding (K/A mutation in the Walker A motif) or hydrolysis (E/Q mutation in the Walker B motif) in specific AAA+ domains. Studies on dynein homodimers showed that ATPase mutations of monomers of a truncated 331-kDa S. cerevisiae dynein (herein referred to as Dyn) at AAA1 fully abolish motility [29] , [30] and AAA3 mutations result in movement tenfold slower than native dynein [29] , [30] . We previously demonstrated that a heterodimer of AAA1 E/Q (E1849Q) and wild-type (WT) monomers walk processively [18] . However, it remained unclear whether the processive motility is facilitated by the ability of the WT monomer to drag its inactive partner, or AAA1 E/Q releases from MT through ATP binding to its AAA1 site. To address this question, we introduced different ATPase mutations to one of the heads of a dynein heterodimer constructed with FRB-FKBP12 tags ( Fig. 1b ; Supplementary Table 1 ) [31] , [32] and tested their motility by total internal reflection fluorescence microscopy. A heterodimer of FRB-Dyn and FKBP12-Dyn (WT/WT) moves at slightly reduced velocity (65±2 nm s −1 , s.e.m.) and processivity (0.8±0.2 μm, 95% confidence interval (CI)) compared with glutathione s-transferase (GST)-Dyn (99±2 nm s −1 and 1.1±0.1 μm, Fig. 1c ), as previously shown [32] . When ATPase mutations were introduced to one of the monomers, both the velocity and processivity of the heterodimer were affected. Compared with WT/WT, velocity and run length of the AAA1 E/Q /WT heterodimer was reduced 20%, while AAA1 K/A /WT motors moved 60% slower and had twofold longer run length ( Fig. 1c,d ). These results indicate that a WT monomer can pull an inactive AAA1 mutant head faster when the mutant head has a reduced MT affinity, at the expense of reduced processivity. AAA3 K/A /WT (K2424A) and AAA3 E/Q /WT (E2488Q) heterodimers showed a similar reduction in motor velocity to AAA1 K/A /WT ( Fig. 1c ), suggesting that ATPase activity at AAA3 may regulate the communication between AAA1 and MT-binding affinity [33] . The velocity of the mutant heterodimers is linearly related to the probability of a processive run ending per unit time ( Fig. 1e ). The WT head can pull its inactive partner faster when it has a reduced MT affinity (for example, AAA1 E/Q ), but these constructs are less processive than those where the mutant head is locked in a state with high affinity to MT. The results suggest that the magnitude of dynein processivity is determined by the duty ratio (the ratio of MT-bound to unbound time in a stepping cycle) of each head, not by the precise coordination of the stepping cycles of the heads through a nucleotide-gating mechanism [19] , [20] . Minimal requirements of dynein processivity To test whether stacking interactions between the AAA+ rings [28] are required for dynein motility, we created a ‘ringless’ dynein monomer in which the AAA+ ring and the linker are replaced with a monomeric seryl-tRNA synthetase (SRS) fused with the dynein stalk and MTBD [34] , [35] . If interaction between the two rings in a dimer must occur at some point in the ATPase cycle, a dynein heterodimer with a single ATPase ring is not expected to move processively. We tested two strongly bound SRS chimeras, one with a full-length dynein-coiled coil (SRS 85:82 ) and a one-quarter-length mutant (SRS 22:19 ) ( Fig. 2a ). Both constructs showed processive, minus-end-directed motion when dimerized to the linker domain of a WT dynein monomer ( Fig. 2b and Supplementary Movie 1 ). Remarkably, SRS 22:19 /WT had a mean velocity and processivity similar to WT/WT, although it lacks the entire AAA+ ring and the linker domain in one head. SRS 85:82 /WT was approximately threefold slower and twofold more processive ( Fig. 2c and Supplementary Fig. 1 ). The difference between the velocities and run lengths of the two constructs may be due to the geometrical constraints imposed by the altered stalk length. High-resolution tracking assays with SRS 85:82 /WT ( Fig. 2d ) showed that SRS 85:82 had similar step-size distribution to the WT dynein monomer ( Fig. 2e ) [18] . The results exclude direct mechanical or allosteric interactions between the two AAA+ rings as a required mechanism for dynein processivity. 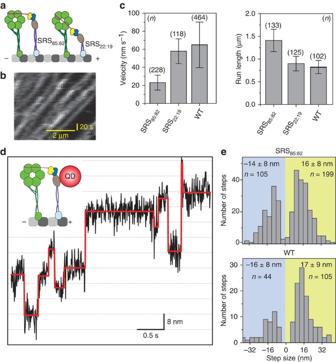Figure 2: Dynein processivity requires a single motor domain. (a) Possible ring–ring communication between the two heads is abolished by replacing one of the monomers with a SRS-MTBD chimera. (b) A kymograph of SRS85:82/WT showing that it moves processively along MTs. (c) The average velocity (±s.d.) and run length (±95% CI) of the SRS-MTBD/WT constructs compared with WT/WT. (d) An example high-resolution tracking trace (black) and stepping fit (red) of the SRS85:82head. (e) Histograms of the step sizes for the SRS (upper) and WT (lower) heads (mean±s.d.). Figure 2: Dynein processivity requires a single motor domain. ( a ) Possible ring–ring communication between the two heads is abolished by replacing one of the monomers with a SRS-MTBD chimera. ( b ) A kymograph of SRS 85:82 /WT showing that it moves processively along MTs. ( c ) The average velocity (±s.d.) and run length (±95% CI) of the SRS-MTBD/WT constructs compared with WT/WT. ( d ) An example high-resolution tracking trace (black) and stepping fit (red) of the SRS 85:82 head. ( e ) Histograms of the step sizes for the SRS (upper) and WT (lower) heads (mean±s.d.). Full size image We hypothesized that the velocity and processivity of the SRS constructs depend on the MT affinity of the SRS-MTBD tether. To test whether a ringless head must maintain a high MT affinity for processive motion, we used a SRS 89:82 construct with an altered coiled-coil registry, which has nearly two orders of magnitude lower MT affinity from SRS 85:82 (ref. 34 ). SRS 89:82 /WT was not able to move unidirectionally, and instead diffused along MTs ( Supplementary Fig. 2 ). The lack of processivity suggests that the inactive MT tether must have sufficient MT affinity to allow processive motion. We next tested whether the velocity of a dynein monomer with a tightly bound SRS 85:82 tether could be increased by reducing the MT affinity of the tether. Addition of up to 100 mM KCl decreased the dissociation constant ( K d ) of the SRS 85:82 -MTBD from MTs by ~30-fold ( Supplementary Fig. 2c ). While the velocity of a WT homodimer remains unaltered by addition of 100 mM KCl, the velocity of the SRS 85:82 /WT increased by 50% ( Supplementary Fig. 2e ), providing further evidence that motor velocity increases by reducing the MT affinity of a strongly bound inactive MT tether ( Fig. 1c,e ). The linker is a mechanical element that powers motility We next tested the mechanism by which the active head can drag its inactive partner forward, presumably via forces generated by the powerstroke of its linker. Although evidence that the linker can power motility was observed in truncated monomeric dyneins [32] , [36] , the role of linker in processive motility and force generation remains unclear. The powerstroke model [9] , [11] suggests that a head that generates force must be attached to the other head through its linker domain, either to push against the other head or to pull it forward. We tested this hypothesis by engineering a heterodimer composed of two catalytically identical but mechanically distinct monomers. The N-terminal linker of one monomer was attached to the C terminus of the other monomer, resulting in a heterodimer of a bound-linker head (BLH) and a free-linker head (FLH) ( Fig. 3a ). According to the powerstroke model, inhibiting the linker swing in the BLH would be predicted to abolish motility, while motors with an inhibited FLH would remain motile. 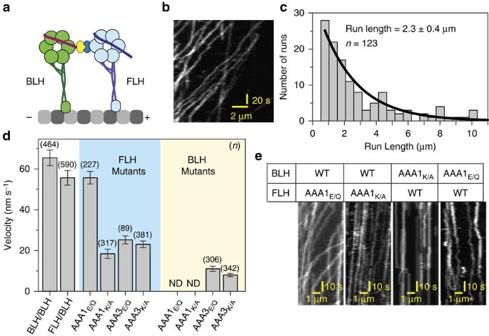Figure 3: The linker provides force to drive the motility of a dynein dimer. (a) Dimerization of the C-terminal ring of one head to the N-terminal tail of the other results in a dimer of a free-linker head (FLH) and a bound-linker head (BLH). (b) Kymograph showing that the FLH/BLH heterodimer is capable of processive motility. (c) Run length histogram of FLH/BLH at 2 mM ATP, with maximum likelihood fit (±95% CI). (d) The average velocities (±s.e.m.) of FLH/BLH constructs carrying an ATPase mutation in either the AAA1 or AAA3 site in one head (ND: motility not detected). (e) Kymographs of ATPase mutants of the FLH or BLH at 2 mM ATP. The AAA1K/Amutation on BLH abolishes directional motility, whereas AAA1E/Qmutation leads to non-directional diffusion along the MT. The same mutations on FLH do not stop motility, indicating that BLH monomer is responsible for FLH/BLH motility. Figure 3: The linker provides force to drive the motility of a dynein dimer. ( a ) Dimerization of the C-terminal ring of one head to the N-terminal tail of the other results in a dimer of a free-linker head (FLH) and a bound-linker head (BLH). ( b ) Kymograph showing that the FLH/BLH heterodimer is capable of processive motility. ( c ) Run length histogram of FLH/BLH at 2 mM ATP, with maximum likelihood fit (±95% CI). ( d ) The average velocities (±s.e.m.) of FLH/BLH constructs carrying an ATPase mutation in either the AAA1 or AAA3 site in one head (ND: motility not detected). ( e ) Kymographs of ATPase mutants of the FLH or BLH at 2 mM ATP. The AAA1 K/A mutation on BLH abolishes directional motility, whereas AAA1 E/Q mutation leads to non-directional diffusion along the MT. The same mutations on FLH do not stop motility, indicating that BLH monomer is responsible for FLH/BLH motility. Full size image Motility assays revealed that the FLH/BLH heterodimer moves processively towards the minus end of MTs at 85% of the velocity of the WT/WT heterodimer ( Fig. 3b and Supplementary Movie 2 ). Intriguingly, the run length of FLH/BLH (2.3±0.4 μm; mean±95% CI) was more than double that of WT/WT ( Fig. 3c ). We next tested the motility of FLH/BLH heterodimers carrying a single AAA1 ATPase mutation [12] . AAA1 mutations to the FLH resulted in similar effects to those observed for the N-terminally dimerized mutant heterodimers: A AAA1 E/Q mutation (FLH AAA1 E/Q /BLH) had a minimal effect on motor velocity, whereas FLH AAA1 K/A /BLH motors suffered a threefold reduction in velocity ( Figs 1c and 3d ). In contrast, introducing the same AAA1 mutations to the BLH (FLH/BLH AAA1 K/A and FLH/BLH AAA1 E/Q ) fully stopped directional motility ( Fig. 3d,e ). While FLH/BLH AAA1 K/A motors remained fixed to a single location on the MT, FLH/BLH AAA1 E/Q showed ATP-dependent non-directional diffusive behaviour along MTs ( Fig. 3e ), consistent with reduced MT affinity of the AAA1 E/Q monomer in the presence of ATP ( Supplementary Fig. 3 ). The AAA3 mutants are able to undergo linker swing [12] , but result in slower motility [31] . Consistently, AAA3 mutations to FLH and BLH moved processively at lower speeds in comparison with WT constructs. Together, the results support that the ATP-dependent linker swing is the force generation mechanism for the motility of a dynein dimer. Tension on the linker gates ATP-dependent MT release We next investigated whether the linker domain has a regulatory role in the dynein stepping mechanism in addition to generating force. High-resolution tracking studies [18] , [19] showed that the two heads of a dynein dimer step independently when they are positioned close to each other on a MT. However, when the heads are separated, the trailing head becomes more likely to step. At high interhead separations, dynein may experience intramolecular tension that favors the release of the trailing head [37] . To investigate whether tension on the linker domain affects the mechanochemical cycle of dynein, we developed an optical trapping assay to measure the nucleotide-dependent MT-release rates under load ( Fig. 4a ). Polystyrene beads were sparsely coated with monomeric dynein and moved ±250 nm between two positions above the MT in a square-wave pattern ( Fig. 4b ). When a WT monomer binds to the MT, the bead is unable to follow the trap to the next position. In this state, the trap exerts a constant force on the motor, depending on the bead-trap separation, until the motor releases from the MT. The assay enables direct measurement of release rate over a large range of forces (0.5–12 pN). A similar approach using an alternate geometry was recently used to measure myosin-unbinding forces [38] . Our assay is a significant improvement compared with previous motor-unbinding assays that measured average rupture force under constantly increasing force [39] , because it better represents the situation in a walking two-headed motor where heads are likely to experience a constant force before releasing from the MT. 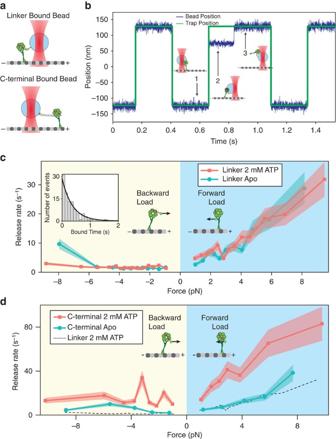Figure 4: Tension on the linker inhibits nucleotide-dependent release of dynein from MTs. (a) Dynein monomers are attached to a polystyrene bead either through the N terminus of the linker via a GFP-antibody linkage, or through the C terminus of the ring via a 74-bp long DNA tether (not to scale). (b) A representative trace showing bead position (blue) and trap position (green). (c) Force-dependent release rates of dynein monomers when the trapped bead is attached to the N-terminal linker domain. The distribution of the forward and backward release rates are unaffected by the presence (red,n=3,003) and absence (blue,n=2,335) of ATP. Shaded regions indicate 95% confidence intervals. Inset: a representative example of the distribution of measured MT-bound times at 0.94 pN average force towards the MT minus-end at 1 mM ATP. Black curve represents maximum likelihood fit to the dwell time histogram. (d) Force-dependent release rates when dynein is pulled through the C terminus. The rate is similar to the N-terminal attachment case (dotted black line) in the absence of ATP (blue,n=1,105), but increases several fold in the presence of 2 mM ATP (red,n=1,652). Figure 4: Tension on the linker inhibits nucleotide-dependent release of dynein from MTs. ( a ) Dynein monomers are attached to a polystyrene bead either through the N terminus of the linker via a GFP-antibody linkage, or through the C terminus of the ring via a 74-bp long DNA tether (not to scale). ( b ) A representative trace showing bead position (blue) and trap position (green). ( c ) Force-dependent release rates of dynein monomers when the trapped bead is attached to the N-terminal linker domain. The distribution of the forward and backward release rates are unaffected by the presence (red, n =3,003) and absence (blue, n =2,335) of ATP. Shaded regions indicate 95% confidence intervals. Inset: a representative example of the distribution of measured MT-bound times at 0.94 pN average force towards the MT minus-end at 1 mM ATP. Black curve represents maximum likelihood fit to the dwell time histogram. ( d ) Force-dependent release rates when dynein is pulled through the C terminus. The rate is similar to the N-terminal attachment case (dotted black line) in the absence of ATP (blue, n =1,105), but increases several fold in the presence of 2 mM ATP (red, n =1,652). Full size image We first pulled dynein monomers from the N-terminal linker domain in the absence of nucleotide. There was a clear difference in the average time a monomer remained bound to the MT, depending on the direction of the applied load. When force was applied towards the MT minus end, the monomers rapidly released from MTs ( Fig. 5c ). In the apo state, the release rate increased from 5 s −1 at 1–2 pN, to 20 s −1 at 5–6 pN ( Fig. 5c ). In contrast, release towards the plus end is significantly slower (~1.5 s −1 ) and independent of load up to 7 pN, the highest measured stall force of native yeast dynein [40] . We observed a similar asymmetry in release of the SRS 85:82 chimera, which contains mouse dynein MTBD ( Supplementary Fig. 3a,c ). The results indicate that dynein favors release towards its natural direction of motion under tension. The asymmetric release of a head is an intrinsic property of its stalk and MTBD, and does not depend on its AAA+ ring or linker. In addition, the preferential release under forward load is not specific to yeast dynein, and may be well conserved in dyneins in higher organisms. 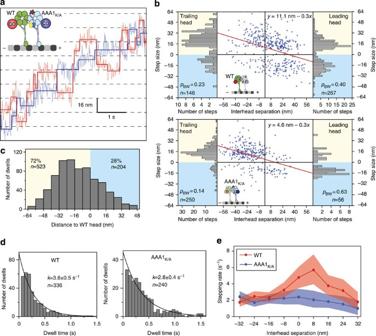Figure 5: Tension gating of a dynein head is observed at high interhead separations in a motile dimer. (a) A representative trace showing simultaneous tracking of AAA1K/A/WT stepping properties with two colours of quantum dots at saturating (1 mM) ATP. (b) The scatter plots represent the step sizes of WT (top) and AAA1K/A(bottom) heads as a function of interhead separation. Interhead separation is positive when the stepping head is in the lead. Slope andyintercept of the linear fit (red line) reveal the change in step size per nm extension between the heads and the net bias to move towards the minus-end, respectively. Both heads take smaller steps when they release the MT in the leading position, similar to native dynein. The AAA1K/Ahead takes mostly backward steps when stepping from the leading position (probability of backward stepping,pBW=0.63). (c) The AAA1K/Ahead remains in the trailing position 72% of the time. Distance to the WT head is positive when the AAA1K/Ahead is in the lead. (d) Histogram of the dwell time between steps of the WT (left) or AAA1K/A(right) head, independent of the action of the other head, with exponential fit (±95% CI). (e) Stepping rates of the WT and AAA1K/Aheads as a function of interhead separation (shaded region is the 95% CI). The WT head steps more frequently when it is positioned close to the AAA1K/Ahead, and is otherwise as a similar rate to the AAA1K/Ahead, indicating that the WT head is gated at high interhead separations. Figure 5: Tension gating of a dynein head is observed at high interhead separations in a motile dimer. ( a ) A representative trace showing simultaneous tracking of AAA1 K/A /WT stepping properties with two colours of quantum dots at saturating (1 mM) ATP. ( b ) The scatter plots represent the step sizes of WT (top) and AAA1 K/A (bottom) heads as a function of interhead separation. Interhead separation is positive when the stepping head is in the lead. Slope and y intercept of the linear fit (red line) reveal the change in step size per nm extension between the heads and the net bias to move towards the minus-end, respectively. Both heads take smaller steps when they release the MT in the leading position, similar to native dynein. The AAA1 K/A head takes mostly backward steps when stepping from the leading position (probability of backward stepping, p BW =0.63). ( c ) The AAA1 K/A head remains in the trailing position 72% of the time. Distance to the WT head is positive when the AAA1 K/A head is in the lead. ( d ) Histogram of the dwell time between steps of the WT (left) or AAA1 K/A (right) head, independent of the action of the other head, with exponential fit (±95% CI). ( e ) Stepping rates of the WT and AAA1 K/A heads as a function of interhead separation (shaded region is the 95% CI). The WT head steps more frequently when it is positioned close to the AAA1 K/A head, and is otherwise as a similar rate to the AAA1 K/A head, indicating that the WT head is gated at high interhead separations. Full size image ATP addition is expected to increase the MT-release rate independent of load [13] . Surprisingly, the release rate profile was unchanged upon addition of 2 mM ATP ( Fig. 4c ). We hypothesized that this could be due to the force being applied to dynein through its linker. To test this possibility, we repeated the trapping assay with the bead bound to the C terminus of a dynein monomer through a short (74 bp) DNA tether ( Fig. 4a ). In the absence of ATP, we observed similar release rates to those of monomers pulled through the linker domain, implying that DNA attachment does not induce changes in the release rate. Remarkably, the release rate increased several fold upon addition of 2 mM ATP ( Fig. 4d ). The results show that tension upon the linker domain inhibits nucleotide-dependent release of dynein from MTs, which may explain the altered stepping behaviour of a dynein dimer at high interhead separations [19] , [20] . Dynein stepping is gated at high interhead separations We next tested whether gating caused by intramolecular tension plays any role in the stepping mechanism of active dynein dimers. If tension on the linker inhibits nucleotide-dependent release from the MT, we expect to observe altered stepping rates at high interhead separations. To experimentally test this effect, we tracked the stepping behaviour of both heads of the AAA1 K/A /WT heterodimer ( Fig. 1b ) at saturating (1 mM) ATP. The AAA1 K/A mutant head could be envisioned as a MT tether in a high-affinity conformation, because it is unable to produce force [13] and remains tightly bound to MT [31] . Therefore, AAA1 K/A can only step when released from MT under tension generated by the linker domain of the WT head. The effects of this mutation were evident in two-colour tracking traces ( Fig. 5a ). The step sizes of both heads negatively correlate with on-axis separation of the heads ( Fig. 5b ), similar to native dynein. However, the net bias to step towards the MT minus end was significantly higher in the WT head than in the AAA1 K/A head (11.1±2.1 versus 4.6±2.2 nm (±95% CI), respectively) when the heads are positioned close to each other. The AAA1 K/A head trails often (72% of dwells) and has a low probability (28%) to take a step when it is in the leading position ( Fig. 5b,c ). The results are consistent with the inability of the AAA1 K/A head to step on its own and the resistance of the MT-binding interface to release under plus-end-directed forces. If the heads are fully uncoordinated, the WT head in the AAA1 K/A /WT heterodimer is expected to have the same stepping rate as a head in a WT/WT homodimer. We observed that the stepping rate of the WT head (3.8±0.5 s −1 ) is significantly higher than the mutant head (2.8±0.4 s −1 , P <0.0001, Kolmogorov–Smirnov test, Fig. 5d ), but it is lower than the MT-stimulated ATPase rate per head (8 s −1 ) in WT/WT [32] . This suggests that the stepping motion of the WT head is slowed by the presence of the mutant head. The analysis of two-colour traces as a function of interhead separation revealed that the stepping of the heads depend on interhead separation. The stepping rate of the AAA1 K/A head was low and slightly decreasing with increased interhead separation ( Fig. 5e ). In comparison, the stepping rate of the WT head (6.0±2.0 s −1 ) was nearly as high as the bulk ATPase rate at low interhead separations [29] , but it is similar to that of AAA1 K/A at high interhead separations ( Fig. 5e ). We concluded that a dynein dimer experiences intramolecular tension through its linker domains at high interhead separations. Tension on the linker gates ATP-dependent stepping of the head from the MT. A model for dynein motility We combined our experimental results and developed a quantitative model for dynein motility. We envisioned that a head can release from the MT either through ATP binding or by tension ( Fig. 6a ). At low separations, the heads are fully uncoordinated. One of the heads binds ATP and takes a step with a rate of 8 s −1 (ref. 32 ). The other head serves as a tether to prevent release of the motor from MT [18] . At high interhead separations, tension on the linkers prohibits release of a head from MT through ATP binding ( Fig. 6a ). In this case, a head releases from MTs under tension and relieves the tension by stepping towards the tethered head. 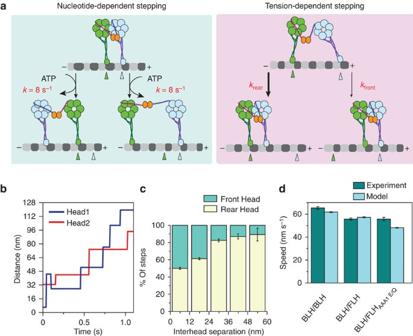Figure 6: A model for dynein motility. (a) Two proposed mechanisms of dynein stepping. (Left) when the heads are close to each other, either head can release the MT and step forward upon ATP binding. (Right) When the heads are far apart, tension on the linker prevents ATP-dependent MT release, and the asymmetry of the release rates under tension favors the trailing head to take a step. (b) A representative Monte Carlo simulation of dynein motility shows stepping of the two head domains (blue and red). (c) The trailing head is more likely to take a step in simulated traces as the interhead separation increases. The data shown are the average of 200 simulations (±s.d.). (d) The average velocity of 200 100-s simulated traces (±s.e.m.) agrees well with measured velocities for various dynein mutants (±s.e.m.,n>100). The results of the model are within ±15% of the experimental data. Figure 6: A model for dynein motility. ( a ) Two proposed mechanisms of dynein stepping. (Left) when the heads are close to each other, either head can release the MT and step forward upon ATP binding. (Right) When the heads are far apart, tension on the linker prevents ATP-dependent MT release, and the asymmetry of the release rates under tension favors the trailing head to take a step. ( b ) A representative Monte Carlo simulation of dynein motility shows stepping of the two head domains (blue and red). ( c ) The trailing head is more likely to take a step in simulated traces as the interhead separation increases. The data shown are the average of 200 simulations (±s.d.). ( d ) The average velocity of 200 100-s simulated traces (±s.e.m.) agrees well with measured velocities for various dynein mutants (±s.e.m., n >100). The results of the model are within ±15% of the experimental data. Full size image We used reported step size [19] , [20] and ATPase rates [30] , [33] , as well as our optical trapping data, to test if our model could accurately capture the behaviour observed in native and mutant forms of yeast dynein. Release rates under tension were inferred from fits to the optical trap data ( Fig. 5 and Supplementary Fig. 4 ). Monte Carlo simulations were used to generate stepping traces of a WT/WT homodimer. Simulated traces ( Fig. 6b ) reproduced uncoordinated stepping patterns, with a significant fraction (33%) of steps in the backward direction [18] , [32] . At high interhead separations, the majority of the steps were taken by the rear head, as observed experimentally ( Fig. 6c ) [18] , [19] . The model estimated that the overall stepping rate per head is 7 s −1 , in agreement with the MT-stimulated ATPase rates. The tension-induced stepping pathway constitutes a significant fraction (32%) of dynein stepping motion. We also tested whether our model could reproduce the observed speeds of dynein motility in response to ATPase mutations and altered dimerization geometry. The stiffness of the linkage between the dynein heads remains unknown; therefore the tension between the heads cannot be directly inferred from the interhead separation. Therefore, we tested a wide range of values for linker stiffness ( Supplementary Fig. 5 ). In simulations of these mutants, optical trap data with C- and N-terminal attachment geometries were used to calculate the tension-induced release rates of FLH and BLH, respectively ( Supplementary Fig. 4 ). In the model, the FLH and AAA1 E/Q -mutant heads release from the MT through ATP binding, but do not undergo a powerstroke ( Supplementary Fig. 3b ). We found that the stiffness of 1 pN per 12-nm extension of the linker agreed most closely with the experimental results ( Fig. 6d and Supplementary Fig. 5 ). The velocities of simulated motors were within ±15% of the measured velocities of mutant heterodimers. This number estimates that, at the highest interhead separations (~36 nm), the heads experience 3-pN tension, equivalent to maximal force production of a single dynein motor (manuscript in preparation). The results show that the tension-induced gating mechanism explains the stepping properties of dynein motility. See Methods for a detailed description of the parameters used in the model. Previous studies have shown that individual dynein motor domains are incapable of processive movement and that dimerization restores processivity [32] . However, it remained unclear whether dynein motility specifically requires both monomers to be catalytically active, dimerized through their N-termini, communicating their nucleotide cycles and mechanically coupling their stepping motions with each other. We engineered dynein’s motile properties in predictable ways, which allowed careful examination of structural and catalytic requirements of dynein processivity. Processivity does not require two catalytically active motor domains. Altering the ATPase activity of a single monomer in dynein heterodimers revealed a strikingly different phenotype from identical mutations to homodimeric constructs [29] , [30] . A hydrolysis-deficient AAA1 mutant heterodimer moved at near-WT velocities. These results differ significantly from similar measurements on a kinesin heterodimer carrying a single ATP hydrolysis [41] or binding [42] mutation, which moves 10–20-fold slower than native kinesin. Consistent with the ability of dynein to move without tight interhead coordination, a single force-generating head is able to drive motility nearly as fast as if both heads retained full ATPase activity, provided its inactive partner has moderate affinity for the MT. Dynein’s unique domain architecture has made it possible to isolate the MT-binding interface from its catalytic core. We showed that N-terminal dimerization is not essential for processive motion and alternative dimerization geometries can achieve increased processivity with a minor reduction in motor velocity. The entire AAA+ ring and linker domains of one head can be replaced with an inert protein retaining the MTBD and part of the stalk. Therefore, dynein motility does not require both AAA+ ring domains, and the partner motor does not need to cycle between weakly and tightly MT-bound states. These results raise the possibility that synthetic processive motors may be engineered from a single polypeptide containing one force-producing head and two MT attachment sites. Our ringless dynein heterodimer also excludes direct mechanical or allosteric interactions between the two AAA+ rings as a required mechanism for processivity or force generation. How could dynein walk processively in the absence of interhead communication? We envision that processivity could arise if the duty ratio of a head is sufficiently high (~0.9) to allow the motor to take 100 steps (the average run length is ~1 μm and the average step size is ~10 nm) before dissociation [18] . The duty ratio of Dictyostelium dynein was estimated to be a minimum of 0.6 by the filament gliding assays [36] . Consistent with this idea, we observed that the processivity of engineered dynein heterodimers is correlated with the MT affinity of the mutant head. A swinging motion of the linker domain was shown to drive the MT gliding ability of dynein monomers [32] , [43] . Engineering of a processive dynein dimer with mechanically distinct monomers allowed us to investigate in depth the function of the linker in dynein’s stepping mechanism. By selectively disrupting the linker swing in FLH and BLH mutants, we present strong evidence that the linker powers the motility of a dynein dimer and its N terminus must be tethered to a second MT-binding site to generate an efficient powerstroke. In addition to its function as a mechanical element, the linker is involved in coupling the nucleotide and mechanical states of the motor domain. Reducing the linker length [32] or mutating the residues on AAA5 that make contact with the linker [8] eliminate most of the MT-stimulated ATPase activity, indicating that contacts between the linker and the ring are essential for ATPase activity. Our observation that force on the linker influences dynein’s ability to release from MT in a nucleotide-dependent manner further highlights the connection between MT affinity and linker conformation [13] . Tension on the linker may disrupt these connections and force the linker to attain a fixed conformation relative to the ring. It is also possible that tension on the linker decouples MT affinity from the ATP hydrolysis cycle, such that ATPase activity remains unabated, but MT affinity is not controlled by the nucleotide state. In this case, dynein monomers would be expected to show similar MT-release rates when pulled through the linker, independent of any ATPase mutations in the ring. However, we observed that AAA1 E/Q monomers have higher release rates than WT monomers when force is applied to the linker domain, implying that the nucleotide state is still coordinated with MT affinity ( Supplementary Fig. 3b,c ). Long-range communication between the catalytic sites and the MTBD can be mediated by a coiled-coil segment extending from AAA5 (refs 44 , 45 ). Since the linker runs across the opposite side of the ring [7] , [8] , it is unlikely that the linker orientation directly affects MT affinity. Instead, we propose that linker configuration is coupled to the catalytic activity of the ring, and indirectly affects the MT affinity. In cells, dynein motor activity is regulated by several associated proteins including the dynactin complex, LIS1, and NUDEL [46] . Lis1 forms a dimer, and directly interacts with both motor domains. Lis1 binding induces a persistent high-affinity MT-bound state and slows down dynein motility [47] , [48] . Our results describing how dynein motility responds to perturbations to one of its two motor domains show that for a dynein dimer to be fully inhibited each monomer must be bound to an inactivating factor. This would alter the response of dynein to cytosolic concentrations of regulatory proteins and allows tuning of dynein speed and processivity at different levels. Indeed, monomeric Lis1 is able to inhibit dynein motility, albeit at significantly higher concentrations than that of Lis1 dimer [48] . During yeast cell division, multiple dynein motors bound to the cell periphery pull MTs in opposite directions across the cell. Proper segregation of nuclei requires dynein motors to remain bound to MTs under high tension. We showed that the dynein MTBD remains attached to MTs under plus-end-directed forces, even in the absence of Lis1. Tension on the linker domain also induces a prolonged MT-bound state by inactivating nucleotide-dependent release from MT. This mechanism may contribute to dynein’s ability to move large intracellular cargos and anchor MTs to the cell cortex under high tension. Construct design and yeast cloning An N-terminal truncated S. cerevisiae cytoplasmic dynein gene ( DYN1 ) encoding amino acids 1219–4093 (predicted molecular weight 331 kD, referred to as Dyn) was used as a template for mutagenesis [32] . Dyn was artificially dimerized through an N-terminal GST tag (GST-Dyn). An N-terminal GFP fusion protein of GST-Dyn (GFP-GST-Dyn) has been shown to move at similar velocity and processivity to that of native yeast dynein [32] . Heterodimeric dynein constructs were obtained by replacing the GST tag of GST-Dyn with an FRB tag on one monomer (FRB-Dyn) and an FKBP12 tag on the other monomer (FKBP12-Dyn). FRB and FKBP12 form a heterodimer in the presence of the small molecule rapamycin [31] . A C-terminal HaloTag (Promega) was used to fluorescently label dynein. FRB-Dyn constructs carrying ATPase mutations, AAA1 E/Q (E1849Q), AAA3 E/Q (E2488Q) and monomeric Dyn AAA1 K/A (K1802A), AAA3 K/A (K2424A) were a generous gift of Ronald D. Vale (UCSF). An N-terminal FRB domain was added to the monomeric K/A mutants. FLH constructs were obtained by inserting an FRB or FKBP12 heterodimerization tag to the C terminus of a Dyn construct carrying the appropriate ATPase mutations [32] . Assays on FRB-BLH dimerized to FKBP12-FLH or with FKBP12-BLH dimerized to FRB-FLH did not show a large difference in motor speed verifying that the speed measurements are not affected by which tag is introduced to C and N terminus of the motor. Chimeric constructs which encode a monomeric Thermus thermophilus SRS and the dynein MTBD at different coiled-coil length and registry were generously provided by Ian Gibbons and Andrew P. Carter [34] . A 4 × (GS)-FKBP12 tag was inserted to the C terminus of SRS. For optical trapping experiments, an enhanced GFP gene was added in place of FKBP12. The SRS construct was additionally tagged with an N-terminal HaloTag for fluorescent labelling. Supplementary Table 1 contains all of the constructs used in this study. Protein expression, purification and labelling Dynein proteins were expressed in yeast and purified as described [32] . Purified protein was stored in dynein loading buffer (DLB; 30 mM HEPES pH 7.2, 2 mM MgCl 2 , 1 mM EGTA, 10% glycerol). Expression and purification of SRS-MTBD mutants were carried out in Escherichia coli , as described [34] . For fluorescent tracking experiments, BLH heads containing a C-terminal HaloTag were labelled with 10 μM tetramethylrhodamine (TMR) HaloTag ligand (Promega) for 1 h on ice during the protein preparation, before washing of the Immunoglobulin G beads (GE Healthcare). SRS chimera MT co-sedimentation assay The SRS chimera MT co-sedimentation assay was carried out in DLB as described [34] . Microscope Single-molecule motility assays were performed on a custom-built objective-type total internal reflection fluorescence microscope, equipped with an inverted microscope body (Nikon Ti-Eclipse) with perfect focusing system, 1.45 NA 60 × microscope objective (Nikon, TIRF Plan Apochromat). The sample was illuminated with 488 and 532 nm solid-state lasers (Coherent) to image GFP and TMR, respectively. BLH-TMR was imaged to record the speed and run length data, except in Supplementary Movie 1 in which SRS-TMR is imaged. FLH-GFP was imaged to confirm motility of the FLH (data not shown). For velocity assays, GST-Dyn motility was recorded with a 2-s exposure time under 5.1 mW 532-nm laser exposure. For run length assays, GST-Dyn motility was recorded under 1.9 mW of 532-nm illumination. Laser power and the image acquisition rate were adjusted for other constructs to keep the average distance travelled by motors (~100 nm per image) and the bleaching decay rate of TMR (0.004 per image) constant. Run length assays were done in buffer containing a final concentration of 75 mM K + . Emitted photons were detected by an electron-multiplied charge-coupled device camera (Andor Ixon, 512 × 512 pixels, 16 μm pixel size). The image was magnified by a tube lens to obtain 129.3 nm effective pixel size, calibrated with a reticle containing 100 lines per mm. Single-molecule motility assays Motility assays were performed as described [32] . Sea urchin axonemes were immobilized on a glass coverslip in a flow chamber constructed with double-sided tape. The chamber was washed with 50 μl of DLB followed by 50 μl of DLB supplemented with 1 mg ml −1 casein, 2 mM DTT (DLBC). In total, 200 pM dynein was then perfused into the chamber in DLBC and allowed to bind to MT for 1 min. The flow cell was then washed with 100 μl of DLBC and 20 μl of imaging buffer (DLBC with 1% β-mercaptoethanol, 2 mM ATP and an oxygen scavenging system consisting of 25 mM protocatechuic acid (PCA), 0.35 mg ml −1 protocatechuate-3,4-dioxygenase, 0.6 mM Trolox [49] ). For assays of FRB-FKBP12 heterodimers, 1 μl of 600 nM rapamycin and a total volume of 2 μl of equimolar amounts of FRB- and FKBP12-tagged monomers were mixed and incubated in DLB for 10 min at room temperature. These constructs were then further diluted in DLBC before introducing the motor to sample chamber. In total, 100 nM rapamycin was added to all assay buffers to maintain the dimerization. We are confident that the motility observed was due to heterodimerization because: (1) under the motor concentrations used, we did not observe motility in the presence of only one type of the FRB- or FKBP12-tagged monomers; (2) processive motility of FRB- and FKBP12-tagged monomers was also not observed in the absence of rapamycin; (3) selective ATPase mutations on BLH and FLH resulted in dramatic changes in dynein motility, depending on which head carried the mutation, which would not be possible if the motors observed were not heterodimers; (4) fluorescently labelled SRS chimeras are observed to be motile when heterodimerized with unlabelled dynein monomers ( Supplementary Movie 1 ). Multicolour tracking of AAA1 K/A /WT was performed at 1 mM ATP and movies were recorded at 15 ms frame rate. Quantum dot labelling, imaging and data analysis of the assay were performed as described [18] . Fluorescent spots of individual quantum dots were localized with a two-dimensional Gaussian tracking algorithm. Trajectories of dyneins were fitted by a custom-written step finder algorithm, based on Schwartz Information Criterion [50] . Optical trapping assay A custom-built optical trap consisting of a 2-W 1,064-nm continuous wave laser (Coherent), a Nikon Ti-Eclipse microscope body and a Nikon 100 × 1.49 NA Plan-Apo objective was used to study force-dependent release of dynein monomers. To apply forces through the N-terminal linker of dynein, GFP-tagged dynein monomers were diluted in DLBC and incubated with carboxylated polystyrene beads (0.86 μm diameter, Invitrogen) coated with a rabbit polyclonal anti-GFP antibody (Covance). Antibody coating of the beads was carried out by EDC-NHS crosslinking (Pierce) [40] . The motor-bead mixture was then diluted tenfold in DLBC with 5 mg ml −1 casein, the PCA/PCD oxygen scavenging system and 2 mM ATP. For the apo condition, ATP was not added to the motor-bead mixture, resulting in residual ATP concentrations of ~40 nM, well below dynein’s K M, ATP of ~26 μM (ref. 29 ). The final bead concentration was 0.1% weight/volume. To record data from single monomers, motors were diluted to a level where we observed 5–15% binding probability during the oscillation of the beads. In total, >90% of the binding events terminated with a single release step, indicative of binding of a single dynein monomer. At tenfold higher motor concentrations, significant increase in multiple release events was observed (data not shown), while no events were observed in the absence of motor. To apply forces through the C-terminal ring domain, dynein monomers with a C-terminal Halo tag were labelled with a short (74 bp) double-stranded DNA strand. Two complimentary DNA strands, one with a 5′-biotin modification (5′-Biotin-TTCGGTCAATACCCGGCGCAGAGCGCTCAGGCGCGAG GTCAACAGAGGGCGGAGGGTGGGCCAGCGCGACCCCG-3′), the other with a 5′-amine modification (5′-AmMC6-GTGTCGGGGTCGCGCTGGCCCACCCTCCGCCCTCTG TTGACCTCGCGCCTGAGCGCTCTGCGCCGGGTATTGAC-3′) (IDT) were hybridized by combining 30 μl of each strand from 100 μM stock with 20 μl of DNA buffer (80 mM NaHCO 3 pH 8.4, 200 mM KCl, 5 mM MgCl 2 ), heating at 90 °C for 20 min, cooling to 25 °C for 40 min. The DNA mixture was then reacted with 160 μM HaloTag NHS ligand (Promega) for 6 h at room temperature and the reaction quenched with 1 μl of 1 M glycine, pH 8.4. DNA was then desalted through G-25 spin columns into DNA buffer. Dynein (~400 μl) was then labelled with the purified HaloTag-DNA-biotin for 6 h on ice, and excess DNA was removed through microtubule bind and release purification [32] . This dynein–DNA–biotin complex was then incubated with streptavidin-coated polystyrene beads (0.86 μm diameter, Invitrogen), as described above. The motor-bead mixture was then diluted in the imaging buffer. Cy5-labelled axonemes were adsorbed to the surface of a flow cell before addition of the bead/dynein mixture. The sample was excited with 633 nm HeNe laser (Melles Griot) and axonemes were visualized with a CCD camera. The trapping beam was steered by two computer-controlled acousto-optical deflectors (AA Electronics) to capture and position floating monodisperse beads. Trap stiffness was calibrated for each sample by fitting the windowed power spectrum of a bead trapped 3 μm above the surface of the coverslip to a Lorentzian curve [51] . The microspheres were trapped by a ~50-mW 1,064-nm laser beam to achieve a spring constant of ~0.05 pN nm −1 . A position-sensitive detector (PSD) was located at the back focal plane to detect microsphere displacement. The PSD data were recorded at 20 kHz for calibration and 5 kHz for data acquisition. The response of the PSD was calibrated in each sample by rapidly scanning the laser across a trapped bead in both x and y directions using the acousto-optical deflectors and fitting the resulting curve to a cubic polynomial. This calibration was repeated once at the surface and once 3 μm into the solution to avoid systematic errors in either experimental data or stiffness calibrations. Trapped beads were positioned over a Cy5-labelled axoneme and oscillated between two positions (±125 nm) along the long axis of the axoneme. Bead-trap separation was monitored in real time to prevent trap oscillations during a binding event. The trap was held steady for 0.25 s after the bead returned to the trap centre, and then moved to the opposite position. Microtubule polarity was determined by imaging Oregon green-labelled kinesin motors, which decorate the plus-end of MTs. GFP-labelled kinesin was used to determine MT polarity in trapping experiments on DNA-tethered dynein monomers, which lack GFP. Strong (three to tenfold) asymmetry was observed in the release rate of both linker- and C-terminal-bound dynein monomers in the presence of ATP (all of 11 axonemes tested, data not shown). The rest of the data were collected by assigning the microtubule polarity, based on the asymmetry in the plus- and minus-end-directed release rates of dynein monomers. Data analysis The kymographs of GFP-tagged dyneins were made in ImageJ. For the run length analysis, we chose molecules that moved at least 4 pixels (~500 nm), began their runs at least 5 μm away from the minus-end of MTs and remain fluorescent for at least 50 frames before the end of the movie. Since the average distance travelled by a motor before photobleaching (25 μm) is much greater than the measured average run length (0.8–2.2 μm), we have not included a correction for photobleaching in our analysis. Such a correction would result in an increase of run length of less than 5%, within the error of our measurement. The mean run length was calculated by maximum likelihood estimation of the exponential decay constant and stated errors are the 95% confidence intervals. In optical trap assays, single-step MT-release events were analysed and rare multiple-step release events were discarded from the data analysis. Force-induced MT-release data were fit with a custom step-finding algorithm. Events showing a dwell time of greater than 2.5 ms were evaluated visually to confirm the binding and release of a single monomer. The applied force to the motor was calculated by trap stiffness and the bead-trap separation vector. Data consisting of applied force and dwell time were sorted by force and binned every 100 data points. The dwell times in each bin were fit to a single exponential decay (see Fig. 4c , inset), and resulting rate constant was plotted with the average force of all the data points in the bin. Errors are the 95% confidence intervals. Changing the bin size did not significantly affect the results (not shown). Stepping rate versus interhead separation ( Fig. 5d ) was calculated by taking the number of steps each motor took in a given range of interhead separation (8-nm wide bins from −36 to 36 nm) and dividing by the total amount of time the motor spent in that range of separation. In total, 95% confidence intervals were calculated by bootstrapping. Larger interhead separations were not considered due to the rarity of steps, <10 per bin, preventing accurate determination of stepping rate. In a WT/WT motor, the rates for each motor fall within the 95% confidence interval of each other at all interhead separations (data not shown). Computational model Monte Carlo simulations were run to generate stepping traces of a WT dynein dimer. The model incorporates parameters from bulk ATPase [29] , [32] , optical trap and stepping measurements [18] , [19] of yeast dynein (see below). The model assumes ATP-dependent steps can occur when the interhead separation is less than 20 nm. The WT head can step in an ATP-dependent manner with a rate k 1 =8 s −1 based on bulk ATPase measurements per head [29] , [32] . The stepping head rebinds the MT at a position randomly chosen from a Gaussian distribution with a mean 8±16 nm (±s.d.) towards the minus-end from its partner head. The 8-nm minus-end-directed bias in step size is provided by the ATP-dependent linker swing mechanism [9] . FLH WT and AAA1 E/Q mutants, which lack the ability to generate a powerstroke, undergo non-productive ATP-dependent stepping with a rate k 2 ~20 s −1 , measured from extrapolation to the force-induced release data at 0 pN force at 1 mM ATP ( Supplementary Fig. 4 ). The stepping head rebinds at a position randomly chosen from a Gaussian distribution centered at its partner head with 0±16 nm (s.d.) step size. Tension-dependent steps occur when the interhead separation is greater than 12 nm. In this mode of stepping, the leading head steps backwards with a constant rate of k 3 , determined from the force-induced release data ( Fig. 4 and Supplementary Fig. 4 ). The trailing head steps with a rate k 4 = mx , where x is the interhead separation in nm. m was calculated from linear fits to the force-induced release data ( Fig. 4 and Supplementary Fig. 4 ). The release rates of FLH and BLH under tension were calculated from force-dependent release data on motors pulled from their C terminus and linker, respectively. Tension-induced stepping rate increases at higher interhead separations due to increase in intramolecular tension. Fixing the release rate to be equal to the rate measured for a 1–3 pN bin of force data at all interhead separations did not significantly affect the speeds of any of the mutants (data not shown). After a tension-based step, the motor rebinds the MT at a position randomly chosen from a Gaussian distribution, 8±16 nm from its partner head in the direction of the initial position of the stepping head. When the heads are between 12 and 20 nm apart, both tension-dependent and -independent steps are possible. At separations higher than 20 nm, the ATP-dependent stepping mechanism is abolished due to the increased tension on the linker domain ( Fig. 4c,d ). Excluding tension-independent steps in this state did not significantly affect the results. Monte Carlo simulations The Python code used in the simulations is available at http://physics.berkeley.edu/research/yildiz/SubPages/code_repository.html . For each dwell of the motor, the tension-based rate for the trailing head was recalculated according to the fit line of the optical trap data, and the assumed stiffness of the linkage between monomers (1/12 pN nm −1 ) ( Supplementary Fig. 5 ). Other rates used in the model are shown in Supplementary Table 2 . For each mutant simulated, 200 simulations were run for 100 s with a time step of 0.005 s to estimate the speed of each construct. In simulations of mutant dyneins, C- and N-terminal pulling data were used to calculate the force-induced release rates of FLH and BLH, respectively. How to cite this article: Cleary, F. B. et al. Tension on the linker gates the ATP-dependent release of dynein from microtubules. Nat. Commun. 5:4587 doi: 10.1038/ncomms5587 (2014).